Effector diversification within compartments of theLeptosphaeria maculansgenome affected by Repeat-Induced Point mutations Fungi are of primary ecological, biotechnological and economic importance. Many fundamental biological processes that are shared by animals and fungi are studied in fungi due to their experimental tractability. Many fungi are pathogens or mutualists and are model systems to analyse effector genes and their mechanisms of diversification. In this study, we report the genome sequence of the phytopathogenic ascomycete Leptosphaeria maculans and characterize its repertoire of protein effectors. The L. maculans genome has an unusual bipartite structure with alternating distinct guanine and cytosine-equilibrated and adenine and thymine (AT)-rich blocks of homogenous nucleotide composition. The AT-rich blocks comprise one-third of the genome and contain effector genes and families of transposable elements, both of which are affected by repeat-induced point mutation, a fungal-specific genome defence mechanism. This genomic environment for effectors promotes rapid sequence diversification and underpins the evolutionary potential of the fungus to adapt rapidly to novel host-derived constraints. Fungi are the most important pathogens of cultivated plants, causing about 20% yield losses worldwide. Such diseases are a major cause of malnutrition worldwide [1] . Their phenotypic diversity and genotypic plasticity enable fungi to adapt to new host species and farming systems and to overcome new resistance genes or chemical treatments deployed in attempts to limit losses to crop yields [2] . Along with such genotypic plasticity, natural or anthropogenic long-distance dispersal of fungi allows the emergence of novel, better-adapted phytopathogens and more damaging diseases. These processes of adaptation are exemplified by Leptosphaeria maculans 'brassicae' (Phyllum Ascomycota, class Dothideomycetes), which causes stem canker (blackleg) of oilseed rape ( Brassica napus ) and other crucifers. This fungus has been recorded on crucifers (mainly cabbages) since 1791, but only began to cause substantial damage to broad acre Brassica species and spread around the world in the last four decades [3] . Other phytopathogens often rapidly cause lesions on plants to ensure asexual reproduction. In contrast, L. maculans shows an unusually complex parasitic cycle with alternating saprotrophy associated with sexual reproduction on stem debris, necrotrophy and asexual sporulation on leaf lesions, endophytic and symptomless systemic growth, and a final necrotrophic stage at the stem base [3] . Some features of filamentous fungal genomes are remarkably constant; for instance, size (20–60 Mb typically about 34 Mb), gene number (10,000–13,000), gene content, intron size and number, and the low content of repeated sequences [4] . Comparative genomic approaches have shown that most of the candidate 'pathogenicity genes' (for example, those encoding hydrolytic enzymes that can degrade plant cell walls, or involved in formation of infection structures) analysed in the last decade in a gene-by-gene approach are shared by saprobes and pathogens [4] . These genes were probably recruited as pathogenicity factors when phytopathogens evolved from saprobes, but they do not account for host range or host specificity of phytopathogens. Such roles are played by 'effector' proteins, which modulate host innate immunity, enable parasitic infection and are generally genus, species, or even isolate-specific [5] , [6] . Such effector genes include those with a primary function as avirulence genes or encoding toxins or suppressors of plant defense. While bacteria produce few effectors (typically <30), which mostly seem to suppress plant innate immunity [7] , hundreds of candidate effectors have been identified in oomycetes [8] , [9] , [10] . In fungi, in contrast, such a catalogue of effectors has only been established to-date in the hemibasidiomycete pathogen of maize, Ustilago maydis , in which many of the effector genes are organized as gene clusters [11] . In L. maculans , the only characterized effectors include a toxic secondary metabolite, sirodesmin PL [12] and the products of three avirulence genes, AvrLm1 , AvrLm6 and AvrLm4-7 , of which at least one, AvrLm4-7 , is implicated in fungal fitness [13] , [14] , [15] . These three avirulence genes show typical features of effector genes; that is, they are predominantly expressed early in infection, encode small proteins predicted to be secreted (SSPs) into the plant apoplast and have no or few matches in databases. Intriguingly, all three are located within large AT-rich, heterochromatin-like regions that are mostly devoid of other coding sequences [13] , [15] . In this paper, we describe the genome of L. maculans . We speculate how the genome, characterized by a distinct division into guanidine–cytosine (GC)-equilibrated and AT-rich blocks of homogenous nucleotide composition, has been reshaped following massive invasion by and subsequent degeneration of transposable elements (TEs). We also predict the repertoire of pathogenicity effectors for the first time in an ascomycete genome and we propose how the unusual genome structure may have led to the diversification and evolution of effectors. General features of the L. maculans genome The haploid genome of strain v23.1.3 of L. maculans 'brassicae' was sequenced using a whole-genome shotgun strategy. This fungus is closely related to Phaeosphaeria (Stagonospora) nodorum , Pyrenophora tritici-repentis and Cochliobolus heterostrophus , as seen in the phylogeny based on sequence analysis of a range of genes ( Supplementary Table S1 ; Fig. 1 ). The genome assembly had a total size of 45.12 Mb, scaffolded into 76 SuperContigs (SCs; 30 large SCs >143 kb; Tables 1 and 2 ; Supplementary Table S2 ). The correspondence of SCs to chromosomes was inferred by a combination of approaches ( Fig. 2 ; Supplementary Figs S1 and S2 ). Conglomerated data are consistent with the presence of 17 or 18 chromosomes, ten of which correspond to single SCs ( Supplementary Fig. S1 ; Supplementary Table S2 ). 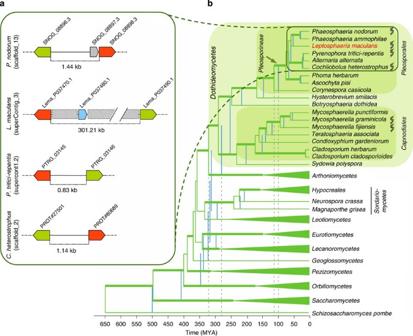Figure 1: Phylogenetic relationships between Dothideomycetes and an example of microsynteny between related species. (a) An example of microsynteny betweenL. maculansand closely related Dothideomycetes,P. nodorum,C. heterostrophusandP. tritici-repentis, showing the integration of an AT-rich genomic region (grey boxes) between two orthologous genes encoding for fungal transcription factors (red and green arrows) of the three other species, along with generation of one novel small-secreted protein-encoding gene (blue arrow) inL. maculansonly. Grey arrow,P. nodorumpredicted gene. The ID of each gene in the corresponding genome sequence is indicated. The intergenic distance (expressed in kb) is shown. (b) A phylogenetic tree and estimated time divergences of major lineages in Ascomycota with a selection of plant pathogenic lineages in Dothideomycetes. The phylogenetic analysis was performed using RaxML44and the chronogram, calibrated using recent data from the literature and fossil dates, produced using r8s (ref.45). Classes outside of the Dothideomycetes were collapsed in TreeDyn, except for Sordariomycetes where the orderHypocrealesrepresented an important calibration point. The blue vertical lines correlate with divergence times when the root of the tree was fixed at 500 MYA, whereas the green lines of the tree represent a fixed root of 650 MYA. The range of dates for the emergence of Dothideomycetes andPleosporineaeare highlighted with stippled lines. Thickened branches on the tree represents nodes that had more than 70% bootstrap values in a RAxML run. Species with genome data are marked with a DNA logo. Figure 1: Phylogenetic relationships between Dothideomycetes and an example of microsynteny between related species. ( a ) An example of microsynteny between L. maculans and closely related Dothideomycetes, P. nodorum , C. heterostrophus and P. tritici-repentis , showing the integration of an AT-rich genomic region (grey boxes) between two orthologous genes encoding for fungal transcription factors (red and green arrows) of the three other species, along with generation of one novel small-secreted protein-encoding gene (blue arrow) in L. maculans only. Grey arrow, P. nodorum predicted gene. The ID of each gene in the corresponding genome sequence is indicated. The intergenic distance (expressed in kb) is shown. ( b ) A phylogenetic tree and estimated time divergences of major lineages in Ascomycota with a selection of plant pathogenic lineages in Dothideomycetes. The phylogenetic analysis was performed using RaxML [44] and the chronogram, calibrated using recent data from the literature and fossil dates, produced using r8s (ref. 45 ). Classes outside of the Dothideomycetes were collapsed in TreeDyn, except for Sordariomycetes where the order Hypocreales represented an important calibration point. The blue vertical lines correlate with divergence times when the root of the tree was fixed at 500 MYA, whereas the green lines of the tree represent a fixed root of 650 MYA. The range of dates for the emergence of Dothideomycetes and Pleosporineae are highlighted with stippled lines. Thickened branches on the tree represents nodes that had more than 70% bootstrap values in a RAxML run. Species with genome data are marked with a DNA logo. Full size image Table 1 Assembly statistics for the L. maculans genome. 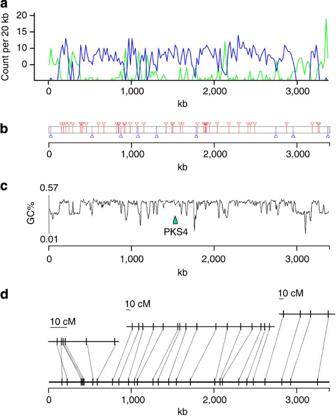Figure 2: Main features of theL. maculansgenome as exemplified by chromosome 5 SuperContig 1. (a) Transposable elements (TEs) distribution and gene density along the supercontig. TE density is drawn in green and gene density is in blue. (b) Location of SSPs (small-secreted protein encoding genes). Blue arrowheads, SSP in AT-blocks, corresponding to TE-rich regions in a; red arrowheads, SSP in GC-blocks, corresponding to gene-rich genome regions in a. (c) GC content along the SC showing alternating GC-equilibrated and AT-rich regions, with location of a polyketide synthase-encoding gene, PKS4. (d) Genetic (upper part, expressed in centiMorgan—cM) to physical (expressed in kb) distance relationship as a function of the isochore-like structure. Lower part: physical location of genetic markers. Upper part of the panel: genetic map using MapMaker/Exp 3.0 with parameters set at likelihood ratio value >3.0 and minimum distance=20 cM. Only markers drawn from the sequence data are represented. Full size table Table 2 Features of genomes of L. maculans and other related Dothideomycetes. Full size table Figure 2: Main features of the L. maculans genome as exemplified by chromosome 5 SuperContig 1. ( a ) Transposable elements (TEs) distribution and gene density along the supercontig. TE density is drawn in green and gene density is in blue. ( b ) Location of SSPs (small-secreted protein encoding genes). Blue arrowheads, SSP in AT-blocks, corresponding to TE-rich regions in a; red arrowheads, SSP in GC-blocks, corresponding to gene-rich genome regions in a. ( c ) GC content along the SC showing alternating GC-equilibrated and AT-rich regions, with location of a polyketide synthase-encoding gene, PKS4. ( d ) Genetic (upper part, expressed in centiMorgan—cM) to physical (expressed in kb) distance relationship as a function of the isochore-like structure. Lower part: physical location of genetic markers. Upper part of the panel: genetic map using MapMaker/Exp 3.0 with parameters set at likelihood ratio value >3.0 and minimum distance=20 cM. Only markers drawn from the sequence data are represented. Full size image Gene models were identified using the EuGene prediction pipeline ( Supplementary Tables S3 and S4 ), and the resulting total of 12,469 genes is consistent with that in other Dothideomycetes ( Table 2 ). 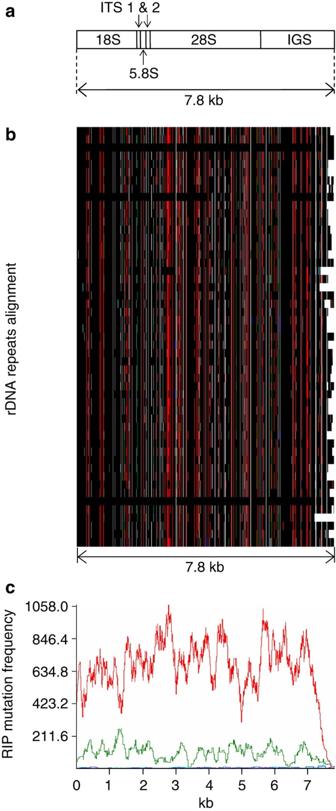Figure 3: Repeat-induced point (RIP) mutation in ribosomal DNA ofL. maculansshown as RIPCAL output. (a) Schematic representation of the rDNA unit inL. maculans(ITS, internal transcribed spacers; IGS, intergenic spacer); (b) a schematic multiple alignment of the 7.8 kb 'complete' ribosomal DNA (rDNA) units occurring in SuperContigs 2 and 19. Polymorphic nucleotides are coloured as a function of the type of RIP mutation observed, with black, invariant nucleotide; red, CpATpA or TpGTpA mutations; dark blue, CpCTpC or GpGGpA mutations; pale blue, CpTTpT or ApGApA mutations; green, CpGTpG or CpGCpA mutations; (c) RIP mutation frequency plot over a rolling sequence window, corresponding to the multiple alignment directly above. Nucleotide polymorphisms (against the alignment consensus, which is also the highest GC-content sequence) mostly correspond to CpATpA or TpGTpA (red curve) and CpGTpG or CpGCpA (green curve). Expression of 84.4% of predicted genes was detected using NimbleGen custom-oligoarrays in free-living mycelium or during early stages of oilseed rape infection ( Table 3 ). About 10% of the genes were significantly overexpressed during infection ( Table 3 ). Taking into account expressed-sequence-tag (EST), transcriptomic, and proteomic support, 84.8% of the gene models were biologically validated ( Table 3 ). The genes are shorter than those in the other Dothideomycetes whose genomes have been sequenced ( Table 2 ). Intergenic distances are shorter than those of P. nodorum , the closest relative to have been sequenced, and bi-directional promoters are common ( Supplementary Table S5 ). Table 3 Comparative features of SSP-encoding genes occurring in diverse genome environments. Full size table Automated finding and annotation of repeated elements in the genome using the REPET pipe-line ( http://urgi.versailles.inra.fr/index.php/urgi/Tools/REPET ) showed that they comprise one-third of the genome compared to 7% in P. nodorum ( Table 2 ). Although most of the repeat elements are truncated and occur as mosaics of multiple families, their origin as TEs is clear ( Supplementary Data S1 and S2 ). Class I elements (see ref. 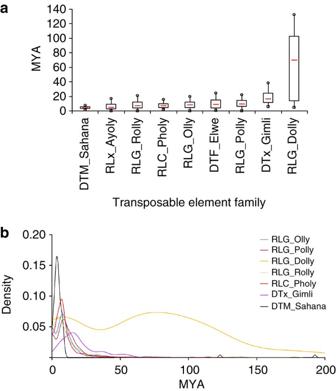Figure 4: Dynamics of transposable elements in theL. maculansgenome. A phylogenetic analysis was used to retrace the evolutionary history of each transposable element (TE) family after elimination of mutations due to repeat-induced point mutations. Terminal fork branch lengths were assumed to correspond to an evolutionary distance used to estimate the age of the last transposition activity. The divergence values were converted to estimated divergence time using a substitution rate of 1.05×10−9substitution per location per year52,53(expressed as 'million years ago' MYA). (a) Box plot graph of divergence times. The red line represents the median value; the boxes include values between the first and the third quartile of the distribution; squares and circles, first and ninth decile, respectively. (b) Kernel density of divergence plots. A R-script was written to plot a histogram of the terminal fork branch length with kernel density estimate for each family. 16 and Table 4 for classification of TEs) dominate with nine families comprising 80% of the repeated elements ( Table 4 , Supplementary Data S1 ). Of these, just four families comprise 11.37 Mb, which is 25% of the genome assembly. Very few, if any, of the TEs are transcribed, as shown by EST inspection and transcriptomic analysis. TEs are clustered in blocks distributed across SCs, and the number of TE copies per SC correlates with size of the SC ( R 2 =0.86; Supplementary Fig. S3 ). Table 4 Main families and characteristics of transposable elements and other repeats in the L. maculans genome. Full size table The TEs are RIP affected Alignment and comparison of repeat families also showed a pattern of nucleotide substitution consisting mainly of C-to-T and G-to-A changes, suggesting the presence of repeat-induced point mutation (RIP). RIP is a premeiotic repeat-inactivation mechanism specific to fungi and has been previously experimentally identified in L. maculans [17] . The L. maculans genome possesses orthologues of all the Neurospora crassa genes currently postulated to be necessary for RIP [18] ( Supplementary Table S6 ). Analysis using RIPCAL, a quantitative alignment-based method [19] , indicated that C bases within CpA dinucleotides were mutated to T, more frequently than the sum of CpC, CpG and CpT dinucleotides, confirming the action of RIP on all of the TEs ( Supplementary Figs S4 and S5 ; Supplementary Data S2 ). The compartmentalized genome of L. maculans The L. maculans genome is larger and has a lower overall GC content (44.1% GC) than those of the related Dothideomycetes P. nodorum , Alternaria brassicicola , C. heterostrophus , P. tritici-repentis or the more divergent species Mycosphaerella graminicola ( Table 2 ). As previously reported for a broader range of fungi [20] , the larger size is consistent with the genome having been extensively invaded by TEs. The GC content of ESTs and other known coding sequences is 50.5%, and the low genome GC content is due to the compartmentalized structure of the genome into GC-equilibrated regions (51.0% GC content, sizes between 1 and 500 kb, average 70.4 kb; henceforth denoted as GC-blocks) alternating with AT-rich regions (henceforth denoted as AT-blocks; averaging 33.9% GC content; with sizes between 1 and 320 kb, average of 38.6 kb). Whole-genome analysis identified 413 AT-blocks and 399 GC-blocks ( Supplementary Table S7 ). The AT-blocks cover 36% of the genome and are distributed within the large SCs, comprising between 23.1 and 49.2% ( Fig. 2c , Supplementary Table S7 ; Supplementary Fig. S6 ). SC22, corresponding to a minichromosome, [21] contains nine AT-blocks amounting to 92.5% of the SC ( Supplementary Table S7 ). As well as differences in GC content, the two types of genomic regions are dissimilar in terms of recombination frequency and gene content. The number of crossovers (CO) along a chromosome ranges between 1.16 and 3.31, depending on size of the chromosome, with one CO every 820 kb on average. The recombination frequency is significantly higher between marker pairs located within GC-blocks than those located on each side of one AT-block ( F -Fisher=5.873, P =0.019; Fig. 2d , Supplementary Fig. S7 ). GC-blocks contain 95% of the predicted genes of the genome, at a higher density (4.2 per 10 kb) than in other Dothideomycetes ( Table 2 ) and are mostly devoid of TEs. In contrast, AT-blocks are gene-poor, comprising only 5.0% of the predicted coding sequences, and mainly contain mosaics of TEs mutated by RIP, thus resulting in a low-GC content of TEs. There are three categories of AT-blocks: telomeres, which include a Penelope retroelement [22] ( Supplementary Fig. S8 ); large AT-blocks (216 sized 13–325 kb); and mid-sized AT-blocks (197 sized 1–13 kb; Supplementary Fig. S9 ), mostly corresponding to single integrations of only two families of DNA transposons ( Supplementary Table S8 ). In almost half of the cases where pairs of orthologues are on the same SC, the genes flanking AT-blocks in L. maculans have orthologues in P. nodorum that are either two consecutive genes or genes separated by only a few others ( Fig. 1a ; Supplementary Data S3 ). A similar pattern was observed for C. heterostrophus and P. tritici-repentis , suggesting that the TEs invaded the genome after the separation of Leptosphaeria from other species of suborder Pleosporineae 50–57 million years ago (MYA; Fig. 1b ). The ribosomal DNA repeat is extensively affected by RIP In eukaryotes, the ribosomal DNA (rDNA) comprises a multigene family organized as large arrays of tandem repeats. The core unit is a single transcription unit that includes the 18S or Small Subunit, 5.8S, and 28S or Large Subunit separated by internal transcribed spacers (ITS1 and ITS2). Each transcription unit is separated by the Intergenic Spacer ( Fig. 3a ). Although essential duplicated regions would be expected to be protected from RIP mutations, the rDNA repeats in L. maculans are in part affected by RIP ( Fig. 3b,c , Supplementary Fig. S10 ). The number of rDNA repeats ranges between 56 and 225 in different L. maculans isolates [23] . The assembly of strain v23.1.3 has >150 repeats, only two of which are highly similar (99.6% identity) and are not affected by RIP. Fifty complete rDNA units and 107 incomplete units are present, and most of them are on extreme ends of SC2 and SC19, which are not complete chromosomes. Many of these repeats are severely affected by RIP ( Fig. 3 , Supplementary Fig. S10 ). Selker [24] has suggested that rDNA repeats in the nucleolus organizer region are protected from RIP. Our data indicate that this is not the case in L. maculans , at least for a part of the array of tandem repeats. Figure 3: Repeat-induced point (RIP) mutation in ribosomal DNA of L. maculans shown as RIPCAL output. ( a ) Schematic representation of the rDNA unit in L. maculans (ITS, internal transcribed spacers; IGS, intergenic spacer); ( b ) a schematic multiple alignment of the 7.8 kb 'complete' ribosomal DNA (rDNA) units occurring in SuperContigs 2 and 19. Polymorphic nucleotides are coloured as a function of the type of RIP mutation observed, with black, invariant nucleotide; red, CpA TpA or TpG TpA mutations; dark blue, CpC TpC or GpG GpA mutations; pale blue, CpT TpT or ApG ApA mutations; green, CpG TpG or CpG CpA mutations; ( c ) RIP mutation frequency plot over a rolling sequence window, corresponding to the multiple alignment directly above. Nucleotide polymorphisms (against the alignment consensus, which is also the highest GC-content sequence) mostly correspond to CpA TpA or TpG TpA (red curve) and CpG TpG or CpG CpA (green curve). Full size image AT-blocks as niches for effectors As described above, AT-blocks have few genes. Furthermore, 76% of these genes are located close to the borders with GC-blocks; only 24% (148 genes) are located within AT-blocks ( Table 3 ; Supplementary Data S4 and S5 ). Protein comparisons and Gene Ontology (GO) analysis indicate that AT-blocks are enriched in genes likely to have a role in pathogenicity ( Supplementary Fig. S11 ). These include orphan genes such as those encoding SSPs, genes involved in response to chemical or biotic stimuli ( Supplementary Fig. S11 ), as well as non-ribosomal peptide synthetases and polyketide synthases, which encode enzymes involved in biosynthesis of secondary metabolites ( Supplementary Tables S9 and S10 ; Supplementary Fig. S12 ). One hundred and twenty-two ( ∼ 20%) of the genes located in AT-blocks encode putative SSPs ( Table 3 ; Supplementary Data S4 ). Only 4.2% of the genes in the GC-blocks encode SSPs (529 genes), and these lack many features of known effectors of L. maculans ( Table 3 ). In contrast, the SSPs encoded in AT-blocks have features indicative of effectors such as low EST support in in vitro grown cultures, low abundance in in vitro secretome samples, increased expression upon plant infection, lack of recognizable domains or homologues in other fungi, and high cysteine content ( Table 3 ; Supplementary Data S4 ). Three TEs, the retrotransposon, RLx_ Ayoly , and two DNA transposons, DTF_ Elwe and DTx_ Gimli , are significantly over-represented in the immediate vicinity of SSPs ( Supplementary Fig. S13 ). Although SSPs are never embedded within a single TE, four SSPs are inserted between two tandemly repeated copies of the DNA transposon DTM_ Sahana . As well as the avirulence genes, two SSPs, LmCys1 and LmCys2, have been functionally analysed. LmCys1 contributes to fungal growth in planta , whereas LmCys2 contributes to suppression of plant defence responses, reflecting their roles as effectors (I. Fudal, unpublished data). Expression of 70.2% of the SSP-encoding genes was detected ( Table 3 ). Of these, 72.7% of the SSP-encoding genes located within AT-blocks (compared with 19.1–22.2% in GC-blocks) were over-expressed at early stages of infection of cotyledons compared with in vitro mycelium growth ( Table 3 ; Supplementary Fig. S14 ). Accordingly, these are postulated to be effectors. In addition, 45% of the predicted SSPs in AT-blocks show a presence/absence polymorphism in field populations, as is the case for avirulence genes in L. maculans and other fungi [25] . The SSPs in GC-blocks include 110 (20.8%) with best BLAST hits to hypothetical proteins from P. nodorum . In contrast, very few SSPs in AT-blocks have identifiable orthologues; only two (1.8%) had a best match to a predicted protein of P. nodorum ( Supplementary Data S4 ). In addition to their lack of orthologues, SSPs in AT-blocks also lack paralogues; only seven genes belong to gene families comprising one to four paralogues. Biases in codon usage occur: in GC-blocks, the preferred codon for each of the 20 amino acids ends with a C or a G and the preferred stop codon is TGA, whereas in SSP genes located in AT-blocks, the preferred codon ends with an A or T for 13 amino acids and the preferred stop codon is TAA ( Supplementary Table S11 ). This, however, only has a limited impact on amino acid favoured usage by SSPs ( Supplementary Table S12 ). Motifs resembling the RxLR translocation motifs of oomycetes were sought [26] following the validation that one such motif, RYWT, present in the N-terminal part of AvrLm6 allows translocation into plant and animal cells [26] . Searches for 〈[RKH] X [LMIFYW] X〉 or 〈[RKH] [LMIFYW] X [RKH]〉 showed that up to 60% of SSPs in AT-blocks and up to 73% of SSP in GC-blocks have putative 'RxLR-like' motifs, implicating these SSPs as candidate effectors that enter plant cells ( Supplementary Data S4 ). History of genome invasion by TEs A range of 278–320 MYA is estimated for the origin of the Dothideomycetes with the crown radiation of the class during the Permian (251–289 MYA; Fig. 1b ). The origins of the plant pathogenic Pleosporineae is determined at 97–112 MYA, placing it in the Cretaceous at a time when flowering plants were beginning to become widespread and eudicots were emerging, during the late Cretaceous and Paleocene. Leptosphaeria likely diverged from the other species analysed between 50 and 57 MYA ( Fig. 1b ). Phylogenetic analyses suggest three main features of genome invasion by TEs: transposition bursts mostly after separation of L. maculans from other species of suborder Pleosporineae as indicated by a 'recent' divergence of the TE families, estimated to 4–20 MYA ( Fig. 4a ); a single or few wave(s) of massive transposition(s) followed by a 'rapid' decay, with some cases like DTM_ Sahana where divergence between copies is extremely low; and no on-going waves of genome invasion by TEs ( Fig. 4b ). Like other organisms with a high density of TEs, the L. maculans genome exhibits 'nesting', where repeats occur within previously inserted TEs. In this fungus, TEs are commonly invaded by other TEs generating a complex 'nesting network'. Eighty-five % of these cases correspond to TEs invading one other TE (primary nesting relationship). Most of the retrotransposon families investigated can invade or be invaded to similar extents ( Supplementary Table S8 ). They also can invade TEs from the same family (self-nests), but usually at a very low frequency compared with invasion of retrotransposons from other families. In contrast, the DNA transposons are more commonly invaded (23.3% of the cases) than acting as invaders (3.5% of the cases; Supplementary Table S8 ). In accordance with overlapping divergence time estimates ( Figs 1b and 4 ), these data indicate periods of overlapping transpositional activity for the long terminal repeats retrotransposons that form the major part of AT-blocks. In such a scenario, the later insertions would be preferentially tolerated in existing decayed transposons. These TEs, having undergone RIP in their turn, would initiate a positive reinforcement loop that would create large AT-rich and gene-poor blocks of homogeneous nucleotide composition. Figure 4: Dynamics of transposable elements in the L. maculans genome. A phylogenetic analysis was used to retrace the evolutionary history of each transposable element (TE) family after elimination of mutations due to repeat-induced point mutations. Terminal fork branch lengths were assumed to correspond to an evolutionary distance used to estimate the age of the last transposition activity. The divergence values were converted to estimated divergence time using a substitution rate of 1.05×10 −9 substitution per location per year [52] , [53] (expressed as 'million years ago' MYA). ( a ) Box plot graph of divergence times. The red line represents the median value; the boxes include values between the first and the third quartile of the distribution; squares and circles, first and ninth decile, respectively. ( b ) Kernel density of divergence plots. A R-script was written to plot a histogram of the terminal fork branch length with kernel density estimate for each family. Full size image The peculiar genomic structure of the L. maculans genome is reminiscent of that discovered in mammals and some other vertebrates: the base composition (GC-content) varies widely along chromosomes, but locally, base composition is relatively homogenous. Such structural features have been termed 'isochores' [27] . In L. maculans , AT-blocks are gene-poor, rich in TEs and deficient in recombination compared with GC-blocks, as in mammals [27] . However, despite these similarities, these genomic landscapes seem to result from different mechanisms. In mammals, the evolution of GC-rich isochores is most likely driven by recombination: genomic regions sized between 100 kb to several Mb with a high recombination rate tend to increase in GC content relative to the rest of the genome. This pattern is not due to a mutational effect of recombination, but most probably due to biased gene conversion [28] . In L. maculans , variations in base composition occur at a much finer scale (the isochore-like blocks are about 10–20 times smaller than in mammals), and it is unknown whether biased gene conversion contributes to increase the GC content of GC-blocks. Conversely, L. maculans isochores can be attributed to the AT-biased mutational pattern induced by RIP mutation of TEs and their flanking regions, thus leading to the evolution of AT-rich isochores. Although the evolutionary forces we postulate shaped the L. maculans genome are common to many species, no fungal genome characterized so far has a similar isochore-like structure. This structure reflects extensive genome invasion by TEs that are nonetheless tolerated by the pathogen and the existence of an active RIP machinery ( Supplementary Table S6 ) that has so far been restricted to the Pezizomycotina subphylum of the Ascomycota and maintenance of sexual reproduction (necessary for RIP). Whereas many species seem to have maintained an active RIP machinery, most of the sequenced fungal genomes are poor in TEs, indicating that run-away genome expansion is normally deleterious. Also, many fungal species have lost the ability to cross in nature (for example, Fusarium oxysporum , Magnaporthe oryzae ) and no case of large-scale sculpting of repeat-rich regions is found in these species, only some ancient signatures of RIP are found [29] . On the basis of the characteristics of avirulence genes in L. maculans , we have described a comprehensive repertoire of putative effectors, which has not previously been done for an Ascomycete. In L. maculans , AT-rich blocks are enriched in effector-like sequences. Location of effector genes has been investigated in only some eukaryotic genomes. A few of the effectors of M. oryzae are subtelomeric [30] , as are those in protozoan parasites of animals, such as Plasmodium and Trypanosoma [31] . Genomes of many Fusarium species contain supernumerary 'B' chromosomes enriched in strain-specific effectors and accounting for the host range of each ' forma specialis ' [32] , [33] . The genome of the oomycete Phytophthora infestans has a plethora of effector candidates embedded in repetitive DNA, and diversification of these effectors is postulated to occur via segmental duplication and variation in intraspecific copy number, resulting in rapidly diverging multigene families [8] . The association between one family of effectors and a LINE in Blumeria graminis , the barley powdery mildew fungus, is proposed to provide a mechanism for amplifying and diversifying effectors [34] . Diversification of effectors in the species mentioned above is postulated to be associated with TE-driven gene duplication and generation of multigene families. In the L. maculans genome, SSP-encoding genes are associated with only a few TE families, which may indicate the ability of TEs to 'pickup and move' effectors. In contrast to the above examples, duplicated effector genes are not present in L. maculans , a finding consistent with the steady inactivation of TEs by RIP and with ancient transposition activity before underdoing RIP. The origins of some effector genes might be at least partially ascribed to lateral gene transfer, a specialty of species within the Pezizomycotina [35] , [36] , [37] . Regardless of the origin of the effector genes, our data suggest that RIP is an important mechanism for generating diversity for genes occurring within AT-blocks of the genome of L. maculans , in a manner not previously documented in any other species. RIP has previously been reported to be restricted to duplicated DNA, but most SSPs or other genes in AT-blocks are present in single copies. How, then, can RIP act on SSP-encoding genes? Studies in N. crassa indicated that the RIP machinery can occasionally overrun the repeated region into adjacent single-copy genes [38] . The embedding of SSPs within RIP-degenerated TEs would then favour such RIP leakage ( Supplementary Fig. S4c ), while selection pressure to maintain functional effectors would prevent them from becoming extinct due to an excessive degree of RIP. This would result in extensive mutation of the affected gene and could account for the mutation rate required for diversifying selection. In contrast, effector genes that became detrimental to pathogen fitness, such as avirulence genes subjected to resistance gene selection, would be lost rapidly as alleles that have undergone extensive RIP are selected for [39] . Evidence for this scenario is provided by examination of RIP indices and in alignment-based studies of alleles of SSPs [39] . The genes (including SSPs) within AT-blocks had higher TpA/ApT indices than those in GC-blocks ( Table 3 ; Supplementary Fig. S15 ), consistent with former genes having been RIP affected. RIP indices for the effectors located within AT-blocks thus would be a compromise between values leading to complete degeneration of the sequence and values enabling sequence diversification while retaining functionality. In plant-pathogen systems, diversifying selection operates on effector genes whose products interact with host proteins [25] . This has been demonstrated for both resistance and avirulence genes, but mechanisms for the diversifying selection of effectors have not been proposed. RIP is shown here to be a potential factor to create the genetic (hyper)variation needed for selection to occur in L. maculans , and this process may also act on effectors in other fungi [40] . These findings allow speculation about an evolutionary scenario for birth of isochore-like structures in the L. maculans genome and its incidence on effector diversification. First, the genome was invaded by a few families of TEs over a (relatively) short time period, mostly after the separation of L. maculans from other related fungi. This TE invasion is unlikely to have been targeted to pre-existing effector-rich genome regions as seen in microsynteny analyses ( Fig. 1a ). Accordingly, the most recent invader, DTM_ Sahana , is not specifically associated with SSPs. Second, waves of overlapping transposition occurred with probable transduction, translation or duplication of genes, resulting in the large amplification of a few families. Such transpositions were primarily targeted to other TEs as shown by the nesting of retrotransposons within other TEs. In parallel, duplicated copies of TEs and genes (either duplicated or not) hosted within TE-rich regions underwent RIP either to extinction for TEs or to generate gene diversity in cases where a strong selection pressure to retain genes was exerted. This eventually resulted in complete inactivation of transposition events, and the sculpting of the genome in an isochore-like structure. Effector genes were maintained in AT-blocks to favour rapid response to selection pressure [39] , [41] and probable epigenetic concerted regulation of their expression ( Supplementary Fig. S14b ). L. maculans shows intriguing evolutionary convergence with both higher eukaryotes in terms of an isochore-like genome structure, and with oomycetes in terms of hosting effectors in highly dynamic 'plastic' regions of the genome [8] . It differs in exploiting a RIP-based mechanism for diversification and inactivation of effector genes. The sequencing of genomes of several species or subspecies of the recent and more ancient outgroups that derived from a common ancestor with L. maculans will provide more information on origin of effectors, genome invasion by TEs and the subsequent effect on generation/diversification of effectors, and thus test the validity of the proposed evolutionary scenario. Phylogenetic analysis A taxon set containing representatives of most classes in Ascomycota was selected from the data matrices produced in two previous papers [42] , [43] . Sequences were concatenated from the Small Subunit and Large Subunit of the nuclear ribosomal RNA genes and three protein coding genes, namely the translation elongation factor-1α and the largest and second largest subunits of RNA polymerase II ( Supplementary Table S1 ). A phylogenetic analysis was performed using RAxML v. 7.0.4 (ref. 44 ) applying unique model parameters for each gene and codon. A combined bootstrap and maximum likelihood (ML) tree search was performed in RAxML with 500 pseudo replicates. The best scoring ML tree was analysed in the program R8sv1.7 (ref. 45 ) to produce a chronogram ( Fig. 1b ). Sequencing and assembly L. maculans 'brassicae' isolate v23.1.3. was sequenced because it harbours numerous avirulence genes, three of which have been cloned by a map-based strategy involving large-scale sequencing of surrounding genomic regions [13] , [15] , [41] . Isolate v23.1.3. results from a series of in vitro crosses between European field isolates [46] and is representative of the populations of the pathogen prevalent in Europe in the mid-1990s. DNA was provided as agarose plugs containing partly digested conidia [21] . Whole-genome shotgun sequencing of three types of libraries (high-copy-number plasmids with 3.3 kb inserts; low-copy-number plasmids with 10 kb inserts and fosmids with inserts 35 or 40 kb; Supplementary Table S13 ) was performed, and also six cDNA libraries, including ones derived from infected plants, were sequenced ( Supplementary Table S14 ). Sequencing reads were assembled using Arachne [47] ( Table 1 ) and the correspondence of SCs to chromosome was inferred by aligning the genetic map to the genome sequence, hybridization of single-copy markers to chromosomal DNA separated by pulsed-field gel electrophoresis, identification of telomere-specific repeats, and by mesosynteny analyses (conserved gene content) with genomes of other Dothideomycetes ( Supplementary Table S2 ). L. maculans genome annotation Automated structural annotation of the genome was performed using the URGI genomic annotation platform, including pipelines, databases and interfaces, developed or locally set up for fungi. The EuGene prediction pipeline v. 3.5a (ref. 48 ), which integrates ab initio (Eugene_IMM, SpliceMachine and Fgenesh 2.6 ( www.softberry.com )) and similarity methods (BLASTn, GenomeThreader, BLASTx), was used to predict gene models. The functional annotation pipeline was run using InterProScan [49] . Genome assembly and annotations are available at INRA ( http://urgi.versailles.inra.fr/index.php/urgi/Species/Leptosphaeria ). Genome assemblies together with predicted gene models and annotations were deposited at DNA European Molecular Biology Laboratory/GenBank under the accession numbers FP929064 to FP929139 (SC assembly and annotations). ESTs were submitted to dbEST under accession nos. FQ032836 to FQ073829. Full description and associated references for sequencing, assembly and gene annotation are provided as Supplementary Methods . Annotation and analysis of repeated elements TEs [16] were identified and annotated using the 'REPET' pipeline ( http://urgi.versailles.inra.fr/index.php/urgi/Tools/REPET ), optimized to better annotate nested and fragmented TEs. Repeats were searched with BLASTER for an all-by-all BLASTn genome comparison, clustered with GROUPER, RECON and PILER, and consensuses built with the MAP multiple sequence alignment program. Consensuses were classified with BLASTER matches, using tBLASTx and BLASTx against the Repbase Update databank [50] and by identification of structural features such as long terminal repeats, terminal inverted repeats [16] and so on. Additional steps of clustering and manual curation of data were performed, resulting in a series of consensuses used as an input for the REPET annotation pipeline part, comprising the TE detection software BLASTER, RepeatMasker and Censor, and the satellite detection softwares RepeatMasker, TRF and Mreps. Analysis of the dynamics of genome invasion by TEs was first based on phylogenetic analysis of each family of repeats, retracing the evolutionary history, regardless of truncation, insertion in other TEs and deletion events [51] . After elimination of all RIP targets, the tree topology was used to retrace the dynamics and demography of TE invasion in the genome. Terminal fork branch lengths from the trees were used to calculate the age of the last transposition events of the copies in the genome. The divergence values were converted in estimated divergence time using a substitution rate of 1.05×10 −9 nucleotide per site per year as applied to fungi [52] , [53] . Dynamics of TE aggregation over time was also analysed by a visual analysis of nesting relationships between TEs. Following the long join annotation, mosaics of TEs were visualised using Artemis v. 12.0 ( http://www.sanger.ac.uk/Software/Artemis/ ) in SC0-22 and a data matrix recording the frequency with which a given TE family was inserted into another one (invader) and the frequency with which one given TE was recipient of an insertion from one or multiple other TEs (invaded TE) was generated ( Supplementary Table S8 ). The statistical identification and significance of the favoured invasion of other TE families as compared with random association was evaluated with a χ 2 -test for given probabilities with simulated P -values, based on 20,000 replicates, as implemented in R. RIP and DeRIP analyses Automated analysis of RIP in L. maculans genomic DNA repeats was performed using RIPCAL ( http://www.sourceforge.net/projects/ripcal ), a software tool that performs both RIP index and alignment-based analyses [19] . In addition, RIP indices such as TpA/ApT and (CpA+TpG)/(ApC+GpT) were used to evaluate the effect of RIP on genes or genome regions for which multiple alignments could not be generated. DeRIP analyses, which predict putative ancient pre-RIP sequences, were performed using an updated version of RIPCAL, including the Perl script 'deripcal' and ripcal_summarise. Analysis of AT-blocks AT- and GC-blocks were manually discriminated from each scaffold using Artemis ( http://www.sanger.ac.uk/Software/Artemis/ ), and a Python script was used to extract sequences and features of AT-blocks. TE content of AT- and GC-blocks was analysed using the REPET pipeline. Size distribution of AT-blocks, occurrence of AT-blocks on chromosomes and relationship between AT-blocks, TE content and chromosome length were calculated. To evaluate meiotic recombination differences between AT- and GC-blocks, micro- and minisatellites located either in GC-blocks or located on both sides of a single AT-block were mapped in a reference cross, and the number of CO between two consecutive markers was calculated. The recombination frequency between two successive markers was calculated, plotted against the physical distance between the two markers and subjected to analysis of variance and a non-parametric test (Mann–Whitney test) using XLStat, to compare recombination frequencies between and within GC-blocks. Intergenic distances were compared between AT- and GC-blocks in L. maculans , and also compared with those of the closely related Dothideomycete, P. nodorum ( Supplementary Table S5 ). GO annotations were compared between genes occurring in AT- and GC-blocks using the blast2GO program. Identification and features of SSPs Non-repeated regions within AT-blocks were identified following masking of TEs with RepeatMasker. The EMBOSS:GETORF program was used on these genomic regions to refine the identification of genes encoding SSPs with a size limit set at 600 amino acids (lower limit: 60 amino acids). A dedicated script combined the outputs of GETORF, FgeneSH and EuGene and a pipeline written in Python screened the predicted proteins according to their size and the presence of signal peptide and transmembrane domains (SignalP 3.0, TargetP and TMHMM). Base composition of the genes encoding SSPs (percent of each base in the sequence, GC content and GC3 content) and amino-acid count of the SSPs (as % of each amino acid in the protein) were calculated by custom Python scripts. Statistical bias in amino acid occurrence was evaluated by an F -test to determine if the variances were equal in both sets, followed by Student's t -test (95% confidence level) to compare the mean use of each amino acid in each set of predicted proteins. Biases in codon usage were evaluated using EMBOSS:CHIPS. A χ 2 -test for given probabilities with simulated values (20,000 replicates) as implemented in R was performed to test random association of SSP-encoding genes in AT-blocks with specific TEs. Motifs similar to the RxLR motif necessary for oomycete effectors to be translocated within plant cells were sought in predicted SSPs, using a Python script aiming at identification of motifs (〈[RKH] X [LMIFYW] X〉 or 〈[RKH] [LMIFYW] X [RKH]〉). Analysis of expression patterns of SSP-encoding genes were compared between in vitro (mycelium grown in axenic medium) and in planta (3, 7 and 14 days after inoculation of oilseed rape cotyledons), either using the L. maculans whole-genome expression array (manufactured by NimbleGen Systems) or by quantitative reverse transcription-PCR on a selected subset of SSP-encoding genes. Acccession codes: Genome assemblies together with predicted gene models and annotations have been deposited in the DNA European Molecular Biology Laboratory/GenBank nucleotide core database under the accession numbers FP929064 to FP929139 (SC assembly and annotations). ESTs were submitted to dbEST under accession numbers FQ032836 to FQ073829. Oligo array data has been deposited in the gene Expression Omnibus under accession code GSE27152 . How to cite this article: Rouxel, T. et al . Effector diversification within compartments of the Leptosphaeria maculans genome affected by repeat-induced point mutations. Nat. Commun. 2:202 doi: 10.1038/ncomms1189 (2011).